Low abundance of the matrix arm of complex I in mitochondria predicts longevity in mice Mitochondrial function is an important determinant of the ageing process; however, the mitochondrial properties that enable longevity are not well understood. Here we show that optimal assembly of mitochondrial complex I predicts longevity in mice. Using an unbiased high-coverage high-confidence approach, we demonstrate that electron transport chain proteins, especially the matrix arm subunits of complex I, are decreased in young long-living mice, which is associated with improved complex I assembly, higher complex I-linked state 3 oxygen consumption rates and decreased superoxide production, whereas the opposite is seen in old mice. Disruption of complex I assembly reduces oxidative metabolism with concomitant increase in mitochondrial superoxide production. This is rescued by knockdown of the mitochondrial chaperone, prohibitin. Disrupted complex I assembly causes premature senescence in primary cells. We propose that lower abundance of free catalytic complex I components supports complex I assembly, efficacy of substrate utilization and minimal ROS production, enabling enhanced longevity. Mitochondria perform vital functions in life such as they provide energy (ATP), generate iron–sulphur clusters, participate in Ca 2+ regulation and have major roles in fatty acid and amino-acid metabolism. They also produce reactive oxygen species (ROS) as metabolic by-products that can damage cellular components and participate in cellular signalling pathways. Mitochondria have long been regarded as crucial in the ageing process. This was originally associated with the (mitochondrial) oxidative stress theory of ageing [1] . However, a recent research has revealed a more complex picture by uncoupling lifespan extension from a decrease in mitochondrial ROS generation or oxidative damage in multiple species [2] , [3] , and other relevant aspects associated with mitochondrial function such as stress responses, apoptosis and cell senescence have also been attracting attention. Mitochondrial biogenesis is an extremely complex process integrating the intra-mitochondrial synthesis of 13 electron transport chain (ETC) proteins coded by the mitochondrial DNA with far more than 1,000 additional proteins that are synthesized in the cytosol as pre-proteins and imported into mitochondria through specific transporters. There are several assembly factors for the ETC, and mitochondrial protein chaperones such as prohibitin (PhB) are thought to be involved in a dynamic balance in the composition of the mitochondriome that determines mitochondrial function [4] . The dynamics of the mitochondriome [5] is further determined by targeted turnover [6] . We aimed to identify in an unbiased approach the proteome composition of mitochondria that might predict longevity in mammals. We reasoned that such a ‘longevity-enabling phenotype’ of mitochondria should be (i) evident in mitochondria from long-living animals at young age (that is, before the death of the first member of the cohort); (ii) common in disparate longevity models and tissues; and (iii) counteracted by ageing. Reduced abundance of ETC proteins and of matrix arm subunits of complex I in particular was found in young mice from long-living mouse cohorts, which was associated with improved complex I assembly, higher state 3 oxygen consumption rates and decreased complex I-linked superoxide production, and was reversed in old mice. Moreover, suppression of complex I assembly decreased mitochondrial oxidative metabolism, increased mitochondrial ROS production and precipitated premature senescence. We suggest that partially assembled matrix arm subcomplexes of complex I, which contain the catalytic subunits, might be detrimental as they only contribute to ROS formation without facilitating electron transport activity and proton pumping. Minimizing the abundance of free catalytic complex I components might be an essential feature of a longevity-enabling mitochondrial phenotype in mammals. Low abundance of ETC complexes associates with longevity To perform an unbiased analysis of mitochondrial protein composition as potential predictor of longevity, we analysed the mouse liver proteome at young age (100% cohort members alive) in two long-lived mice models: the ICRFa strain, a C57Bl/6 substrain [7] with significantly extended longevity under standard ad libitum (AL)-fed condition ( P =0.017; Fig. 1a ); and C57Bl/6 subjected to dietary restriction (DR, 60% of AL food intake) from 3 months of age onwards. DR significantly extended lifespan beyond both AL C57Bl/6 (log-rank test, P =0.0073) and AL ICRFa mice ( P =0.0085; Fig. 1a ). We addressed ageing-related changes by comparing young (7–8 months) and old (30–32 months) ICRFa mice. DR mice were significantly lighter than the AL C57Bl/6, AL ICRFa and old ICRFa mice, whereas there were no differences in body weights among the non-DR mice groups (analysis of variance, P =0.05; Supplementary Fig. 1 ). Food intake was not different between AL ICFRa and AL C7Bl/6 mice, suggesting that the extended lifespan in ICRFa mice is not caused by a concealed DR effect. 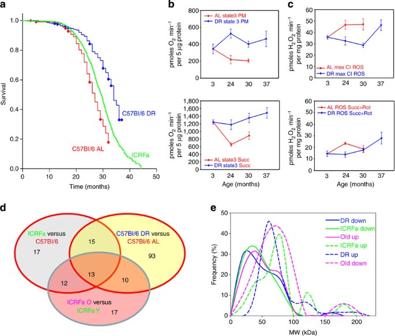Figure 1: Longevity and liver mitochondrial function in male long-living mice. (a) Kaplan-Meier survival curves (right censored) of male C57Bl/6 (red) and ICRFa (green) mice under ad libitum (AL) feeding and of C57Bl/6 mice under 40% DR from an age of 3 months onwards (blue). Group sizes were (censored events in brackets): C57Bl/6 AL 310 (172), C57Bl/6 DR 241 (157) and IRCFa 2391 (1,061). (b) State 3 oxygen consumption rates of purified liver mitochondria from C57Bl/6 mice under AL and DR, respectively, with pyruvate/malate (top) and succinate (bottom) as substrate. Data are mean±s.e.m.,n=4 animals per group. (c) H2O2release from purified liver mitochondria from C57Bl/6 mice under AL and DR, respectively. Data are mean±s.e.m.,n=4. Top: pyruvate/malate plus rotenone, indicating maximum ROS production from complex I (CI). Bottom: succinate plus rotenone, indicating ROS production from sites other than complex I. (d) Numbers of confidently changed proteins in all comparisons. (e) Molecular mass distributions for differentially enriched proteins under DR (blue), in young ICFRa (green) and in old ICRFa (pink). Figure 1: Longevity and liver mitochondrial function in male long-living mice. ( a ) Kaplan-Meier survival curves (right censored) of male C57Bl/6 (red) and ICRFa (green) mice under ad libitum (AL) feeding and of C57Bl/6 mice under 40% DR from an age of 3 months onwards (blue). Group sizes were (censored events in brackets): C57Bl/6 AL 310 (172), C57Bl/6 DR 241 (157) and IRCFa 2391 (1,061). ( b ) State 3 oxygen consumption rates of purified liver mitochondria from C57Bl/6 mice under AL and DR, respectively, with pyruvate/malate (top) and succinate (bottom) as substrate. Data are mean±s.e.m., n =4 animals per group. ( c ) H 2 O 2 release from purified liver mitochondria from C57Bl/6 mice under AL and DR, respectively. Data are mean±s.e.m., n =4. Top: pyruvate/malate plus rotenone, indicating maximum ROS production from complex I (CI). Bottom: succinate plus rotenone, indicating ROS production from sites other than complex I. ( d ) Numbers of confidently changed proteins in all comparisons. ( e ) Molecular mass distributions for differentially enriched proteins under DR (blue), in young ICFRa (green) and in old ICRFa (pink). Full size image We studied liver mitochondrial function in C57Bl/6 during ageing in both AL- and DR-fed mice. Oxygen consumption rates under phosphorylating condition (state 3) using either a complex I-linked substrate (pyruvate plus malate) or a complex II-linked substrate (succinate; Fig. 1b ) progressively declined with age in AL mice but were maintained under DR up to an age of 37 months, that is, beyond the maximum lifespan of the AL mice. Hydrogen peroxide release from complex I was higher under AL than under DR up to an age of 30 months. However, DR only postponed the age-dependent increase and did not prevent it: DR mice at 37 months of age (that is, at equivalent survival rate to 30-month-old AL mice) showed hydrogen peroxide release from complex I as high as AL mice at 30 months ( Fig. 1c ). There were only minor differences in hydrogen peroxide release from sites other than complex I ( Fig. 1c ). In a comparison between ICRFa and C57Bl/6 mice, longer lifespan in ICRFa was also associated with lower hydrogen peroxide release from complex I in isolated liver and brain mitochondria ( Supplementary Fig. 2 ). Proteomic analysis was performed in two separate 6-plex tandem mass tag (TMT) labelling experiments using one-pooled sample in each for cross-standardization. After imposing a 1% false discovery rate (FDR) filter, we identified 7,047 and 6,704 peptides in the two experiments, respectively, and quantified a total of 631 proteins (531 and 497 proteins per experiment) ( Supplementary Data 1–3 ). This represents about half of the mouse mitochondrial proteins in the MitoCarta database and is similar to published data [4] . The molecular weight distribution of the identified proteins mirrored that of all mitochondrial proteins according to the MitoCarta and MitoMiner [8] databases ( Supplementary Fig. 3 ). Our analysis quantified 57 out of the 96 known mouse ETC proteins, namely 67% of complex I proteins, 50% of complex II, 63% of complex III, 46% of complex IV and 76% of complex V. One-hundred seventy-seven proteins showed confidently different abundances in at least one of the three comparisons performed ( Supplementary Data 1–3 ). The number of differentially abundant proteins was the largest (131 proteins) in the AL–DR comparison in C57Bl/6 mice, whereas there were only 57 and 52 differentially abundant proteins for the young C57Bl6–ICRFa and the young–old ICRFa comparisons, respectively ( Fig. 1d ). In general, proteins that were less abundant in the longevity models (and more abundant in old mice livers) tended to be smaller than those that were more frequent in long-living mice ( Fig. 1e ). Out of the 13 proteins that were different in abundance in all three comparisons ( Fig. 1d ), 12 were possibly implicated with longevity because they were less abundant in both longevity models. Moreover, 11 of them were increased in old mice ( Supplementary Table 1 ), together suggesting that low abundance of these proteins at a relatively young age by either genetic or environmental manipulation might predispose to longevity. These proteins included both PhB and PhB 2, and the majority (8 out of 13) were components of the ETC (complexes I, III and V; Supplementary Table 1 ). To identify the functional traits of liver mitochondria associated with longevity, we performed mitochondria-specific KEGG pathway enrichment analysis based on the proteins that were more abundant in liver mitochondria from young C57Bl/6 mice under DR in comparison with AL. 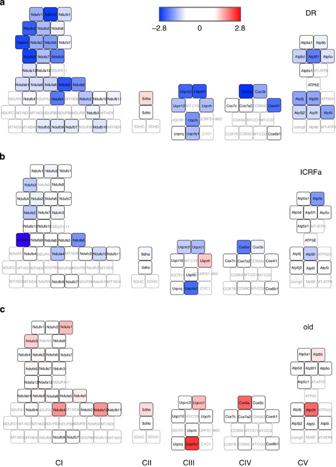Figure 2: ETC proteins are less abundant in long-living mice and increase in old mice. Heatmaps show changes in abundance of all ETC proteins in the comparisons young DR versus young AL C57Bl/6 (a), young ICRFa versus young C57Bl/6 (b) and old versus young ICRFa (c). CI and CV reach out from the inner membrane into the matrix space (upward). Grey symbols represent proteins not identified; and black/white symbols represent abundance that is not significantly changed. Colours indicate fold change. A wide range of diverse metabolic pathways, notably those associated with the Krebs cycle and fatty acid and amino-acid metabolism, was enriched under DR ( Supplementary Table 2 ). However, few of these pathways were similarly enriched in young long-living ICRFa mice or were depleted in old mice. Not a single pathway changed consistently in all three comparisons ( Supplementary Table 2 ), indicating that most of the metabolic pathways that are more abundant under DR are not general longevity-assurance mechanisms. 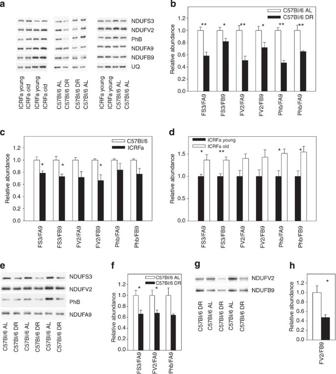Figure 3: Lower abundance of complex I matrix subunits in long-living mice. All data are mean±s.e.m. from four animals per group, *P<0.05, **P<0.01 (t-test). (a) SDS–PAGE western blots of complex I matrix arm subunits NDUFS3 and NDUFV2, PhB and membrane arm subunits NDUFA9 and NDUFB9 in liver mitochondria. Each sample is from a different animal. (b) Relative abundance of matrix subunits NDUFS3 and NDUFV2 and PhB to membrane subunits NDUFA9 and NDUFB9 in liver mitochondria from 7–8-month-old C57Bl/6 mice under AL (open bars) and DR (filled bars). (c) As inb, comparing long-lived ICRFa mice (filled bars) with control C57Bl/6 (open bars) at 7–8 months of age. (d) As inb, comparing young (filled bars) to old (open bars) ICRFa liver mitochondria. (e) SDS–PAGE western blots of the indicated proteins in brain mitochondria. (f) Relative abundance of matrix subunits NDUFS3 and NDUFV2 and PhB to the membrane subunit NDUFA9 in brain mitochondria from 15-month-old C57Bl/6 mice under AL (open bars) and DR (started at 3 months of age, filled bars). (g) SDS–PAGE western blots of the indicated complex I subunits in skeletal muscle mitochondria. (h) Relative abundance of matrix subunit NDUFV2 to the membrane subunit NDUFB9 in muscle mitochondria from 15-month-old C57Bl/6 mice under AL (open bar) and DR (filled bar). In contrast, there were only nine KEGG pathways significantly enriched in an analysis based on proteins less abundant in DR ( Supplementary Table 3 ). Importantly, the four highest ranking of these were also significantly enriched in an analysis based on less abundant proteins in young ICRFa mice ( Supplementary Table 3 ) and equally so in an analysis based on proteins more abundant in old animals ( Supplementary Table 3 ). These four pathways (oxidative phosphorylation, Parkinson’s disease, Huntington’s disease and Alzheimer’s disease) include high proportions of ETC proteins, suggesting that multiple ETC proteins within liver mitochondria are reduced at young age in a longevity phenotype but increased with age. As we were able to quantify the majority of ETC proteins, we examined the changes of the individual ETC subunits in all three comparisons in detail ( Fig. 2a–c ). The abundance of numerous subunits of complexes I, III, IV and V (but not of complex II) was reduced in both long-lived mouse models, which was generally reversed in old mice ( Fig. 2a–c ). There was no evidence for an induction of a mitochondrial unfolded protein response in the long-lived mice with low ETC abundance: several mitochondrial heat-shock proteins (HSPD1, HSPA9 and DSPE1) and the Clpp1 protease were not changed in any of comparisons, whereas heat-shock proteins HSPA5 and HSP90D1 were decreased under DR ( Supplementary Data 1–3 ). Figure 2: ETC proteins are less abundant in long-living mice and increase in old mice. Heatmaps show changes in abundance of all ETC proteins in the comparisons young DR versus young AL C57Bl/6 ( a ), young ICRFa versus young C57Bl/6 ( b ) and old versus young ICRFa ( c ). CI and CV reach out from the inner membrane into the matrix space (upward). Grey symbols represent proteins not identified; and black/white symbols represent abundance that is not significantly changed. Colours indicate fold change. Full size image Low abundance of CI matrix subunits in long-lived mice Strikingly there was a highly skewed pattern of protein abundance changes within complex I. Reduced abundance of complex I subunits in both long-living mice models occurred almost exclusively in subunits localized in the matrix arm while membrane arm subunits were hardly affected ( Fig. 2a,b ). This pattern was partially reversed in the aged mice ( Fig. 2c ). The abundances of PhB and PhB 2, which function as chaperones for ETC proteins and/or as structural scaffolds, paralleled the changes in matrix arm subunits with strong statistical confidence and large fold differences ( Supplementary Table 1 ). We confirmed these observations in a series of SDS–PAGE western blot experiments, by measuring the ratios of selected matrix subunits (NDUFS3 and NDUFV2) and PhB to the membrane subunits NDUFB9 and NDUFA9, which is located at the junction between membrane and matrix arm and is involved in stabilizing this junction [9] ( Fig. 3a ). In agreement with the proteomics results, we found a decreased ratio of matrix subunits and PhB to membrane subunits under DR ( Fig. 3b ) and in liver mitochondria from young long-lived ICRFa mice ( Fig. 3c ), which was reversed in aged liver mitochondria ( Fig. 3d ). Figure 3: Lower abundance of complex I matrix subunits in long-living mice. All data are mean±s.e.m. from four animals per group, * P <0.05, ** P <0.01 ( t -test). ( a ) SDS–PAGE western blots of complex I matrix arm subunits NDUFS3 and NDUFV2, PhB and membrane arm subunits NDUFA9 and NDUFB9 in liver mitochondria. Each sample is from a different animal. ( b ) Relative abundance of matrix subunits NDUFS3 and NDUFV2 and PhB to membrane subunits NDUFA9 and NDUFB9 in liver mitochondria from 7–8-month-old C57Bl/6 mice under AL (open bars) and DR (filled bars). ( c ) As in b , comparing long-lived ICRFa mice (filled bars) with control C57Bl/6 (open bars) at 7–8 months of age. ( d ) As in b , comparing young (filled bars) to old (open bars) ICRFa liver mitochondria. ( e ) SDS–PAGE western blots of the indicated proteins in brain mitochondria. ( f ) Relative abundance of matrix subunits NDUFS3 and NDUFV2 and PhB to the membrane subunit NDUFA9 in brain mitochondria from 15-month-old C57Bl/6 mice under AL (open bars) and DR (started at 3 months of age, filled bars). ( g ) SDS–PAGE western blots of the indicated complex I subunits in skeletal muscle mitochondria. ( h ) Relative abundance of matrix subunit NDUFV2 to the membrane subunit NDUFB9 in muscle mitochondria from 15-month-old C57Bl/6 mice under AL (open bar) and DR (filled bar). Full size image The low relative abundance of matrix subunits of complex I in long-lived mice was not confined to liver. Ratios of matrix subunits NDUFS3 and NDUFV2 to membrane subunit NDUFA9 (as well as PhB/NDUFA9) were indeed lower in brain mitochondria from 15-month-old mice that were subjected to DR from 3 months of age ( Fig. 3e,f ). Similarly in skeletal muscle mitochondria, matrix subunit NDUFV2 showed a decreased abundance in relation to membrane subunit NDUFB9 in DR compared with controls ( Fig. 3g,h ). To see whether the observations made so far are valid in further longevity models, we examined brain and liver mitochondria from mice fed with rapamycin for 4 months. Rapamycin, an inhibitor of the TOR (target of rapamycin) nutrient sensing pathway, is known to extend lifespan in mice [10] . Liver ( Fig. 4a ) and brain ( Fig. 4e ) mitochondria from rapamycin-fed mice did not show altered state 3 oxygen consumption rates nor respiratory control ratio, but hydrogen peroxide release from complex I from both tissue mitochondria was lower ( Fig. 4b,f ). Importantly, ratios of matrix subunits (NDUFS3 and NDUFV2) as well as PhB to membrane subunits (NDUFA9 and NDUFB9) were generally lower in rapamycin-fed animals than in controls in both liver ( Fig. 4c,d , see Supplementary Fig. 4 for uncropped scans) and brain ( Fig. 4g,h ) mitochondria. Thus, a shift to lower abundance of complex I matrix subunits is associated with lower hydrogen peroxide release and a longevity phenotype in multiple tissues and multiple models of longevity. 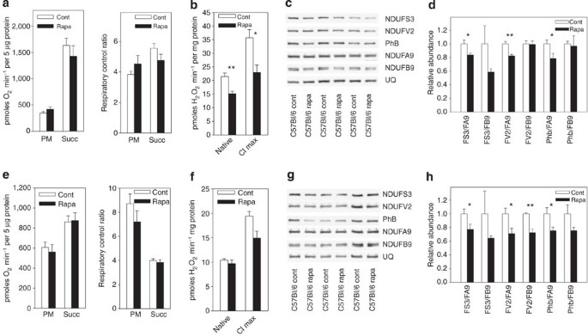Figure 4: Rapamycin treatment reduces ROS production and complex I matrix arm components. All data are mean±s.e.m., 4–5 animals per group, *P<0.05, **P<0.01 (t-test). (a–d) Liver mitochondria from control (Cont) and rapamycin (Rapa)-treated mice. (a) Oxygen consumption rates with pyruvate/malate (PM) or succinate (Succ) as substrate. Left: state 3 respiration rates; and right: respiratory control ratios. (b) H2O2release under native conditions using PM without inhibitors (native) and under PM+rotenone (CI max). (c) SDS–PAGE western blots of complex I matrix arm subunits NDUFS3 and NDUFV2, prohibitin (PhB), membrane arm subunits NDUFA9 and NDUFB9 and UQCRC2 (UQ), a complex III subunit as complex I-independent reference. Please seeSupplementary Fig. 4for uncropped scans of the blots. (d) Relative abundance of matrix subunits NDUFS3 and NDUFV2 and PhB to membrane subunits NDUFA9 and NDUFB9. (e–h) Same asa–d, but from brain mitochondria. Figure 4: Rapamycin treatment reduces ROS production and complex I matrix arm components. All data are mean±s.e.m., 4–5 animals per group, * P <0.05, ** P <0.01 ( t -test). ( a – d ) Liver mitochondria from control (Cont) and rapamycin (Rapa)-treated mice. ( a ) Oxygen consumption rates with pyruvate/malate (PM) or succinate (Succ) as substrate. Left: state 3 respiration rates; and right: respiratory control ratios. ( b ) H 2 O 2 release under native conditions using PM without inhibitors (native) and under PM+rotenone (CI max). ( c ) SDS–PAGE western blots of complex I matrix arm subunits NDUFS3 and NDUFV2, prohibitin (PhB), membrane arm subunits NDUFA9 and NDUFB9 and UQCRC2 (UQ), a complex III subunit as complex I-independent reference. Please see Supplementary Fig. 4 for uncropped scans of the blots. ( d ) Relative abundance of matrix subunits NDUFS3 and NDUFV2 and PhB to membrane subunits NDUFA9 and NDUFB9. ( e – h ) Same as a – d , but from brain mitochondria. Full size image Assembly of complex I is more complete in long-lived mice Mitochondrial complex I is assembled in multiple stages [11] . In HEK293 cells at steady state, complex I subunits exist in a dynamic equilibrium between subcomplexes, the fully assembled holocomplex and supercomplexes [12] , [13] . We hypothesize that relatively lower abundance of matrix to membrane arm components might shift this equilibrium towards less abundant subcomplexes and more fully assembled holocomplex, thus be associated with tighter control of complex I assembly. To test this possibility, we examined the complex I assembly status in liver mitochondria under DR using blue native (BN) gel electrophoresis followed by western blotting ( Fig. 5a ). Complex I activity was preferentially found at the level of fully assembled complex I. Multiple weak activity bands were visible both at supercomplex level and at lower molecular weights ( Fig. 5a,c,e ); however, the sensitivity of the in-gel assay was not sufficient to quantify differences between cohorts. Western blotting of BN gels revealed differential fractions of the tested subunits in smaller subcomplexes ( Fig. 5a ). In DR mitochondria, relative amounts of all subunits in the partially assembled complexes tended to be lower than in AL mitochondria, and this was significant for both matrix arm subunits and for NDUFA9 ( Fig. 5b ). In contrast, complex II activity and the relative amount of the complex II enzyme SHDA was unchanged ( Fig. 5a,b ). 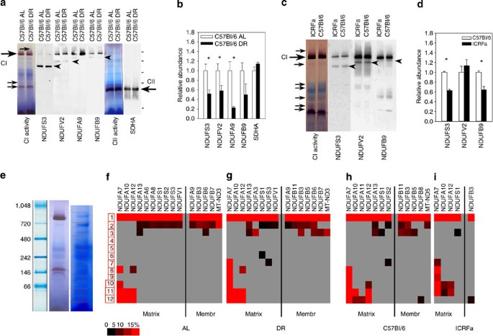Figure 5: Efficient complex I assembly in long-living mice. (a) BN gels/western blots of the indicated subunits of complexes I and II in mice liver mitochondria from 8-month-old mice under AL and DR. Large arrows mark positions of complex I and II holocomplexes. Small arrows indicate positive bands on the complex I activity gel. Arrowheads mark the positions of subcomplexes quantified inb. (b) Normalized ratios of subcomplex/holocomplex band intensity (complex I subunits) or relative intensity (SDHA) on BN gel western blots. Data are mean±s.e.m. from four animals per group, *P<0.05,t-test. (c) BN gels/western blots of the indicated subunits of complex I in mice liver mitochondria from 8-month-old ICRFa and C57Bl/6 mice. The large arrow marks the position of complex I holocomplex, small arrows indicate positive bands on the complex I activity gel. Arrowheads mark the positions of subcomplexes quantified ind. (d) Normalized ratios of subcomplex/holocomplex band intensity on BN gel western blots. Data are mean±s.e.m. from four animals per group, *P<0.05,t-test. (e) Molecular weight marker positions (in kDa), activity gel and BN gel of isolated mouse liver mitochondria indicating the position of slices for proteomic profiling. (f–i) Heatmaps showing the abundance of all identified complex I subunits in slices 2–12 (normalized peptide counts relative to that in the holocomplex (slice 1)). Data are means from three animals per group. (f) C57Bl/6 mice at 15 months of age, AL; (g) C57Bl/6 mice at 15 months of age, DR for 12 months; (h) C57Bl/6 mice at 8 months of age; and (i) ICRFa mice at 8 months of age. Matrix…complex I matrix arm subunits, Membr…complex I membrane arm subunits. Figure 5: Efficient complex I assembly in long-living mice. ( a ) BN gels/western blots of the indicated subunits of complexes I and II in mice liver mitochondria from 8-month-old mice under AL and DR. Large arrows mark positions of complex I and II holocomplexes. Small arrows indicate positive bands on the complex I activity gel. Arrowheads mark the positions of subcomplexes quantified in b . ( b ) Normalized ratios of subcomplex/holocomplex band intensity (complex I subunits) or relative intensity (SDHA) on BN gel western blots. Data are mean±s.e.m. from four animals per group, * P <0.05, t -test. ( c ) BN gels/western blots of the indicated subunits of complex I in mice liver mitochondria from 8-month-old ICRFa and C57Bl/6 mice. The large arrow marks the position of complex I holocomplex, small arrows indicate positive bands on the complex I activity gel. Arrowheads mark the positions of subcomplexes quantified in d . ( d ) Normalized ratios of subcomplex/holocomplex band intensity on BN gel western blots. Data are mean±s.e.m. from four animals per group, * P <0.05, t -test. ( e ) Molecular weight marker positions (in kDa), activity gel and BN gel of isolated mouse liver mitochondria indicating the position of slices for proteomic profiling. ( f – i ) Heatmaps showing the abundance of all identified complex I subunits in slices 2–12 (normalized peptide counts relative to that in the holocomplex (slice 1)). Data are means from three animals per group. ( f ) C57Bl/6 mice at 15 months of age, AL; ( g ) C57Bl/6 mice at 15 months of age, DR for 12 months; ( h ) C57Bl/6 mice at 8 months of age; and ( i ) ICRFa mice at 8 months of age. Matrix…complex I matrix arm subunits, Membr…complex I membrane arm subunits. Full size image Similarly, in a comparison of ICRFa and C57Bl/6 liver mitochondria, relative amounts of NDUFS3 and NDUFB9 in the subcomplexes were lower in the long-lived strain ( Fig. 5c,d ). Longer exposure of the same blots showed incorporation of NDUFS3, NDUFV2 and NDUFB9 into multiple subcomplexes that overlap with bands of weak complex I activity ( Supplementary Fig. 5A ). Even in these low-molecular-weight subcomplexes, less NDUFS3 and NDUFB9 was incorporated in the long-lived ICRFa strain ( Supplementary Fig. 5B ). To assess the distribution of complex I subunits between the holoenzyme and subcomplexes more comprehensively, we performed complexome profiling in mouse liver mitochondria [13] . BN gels were cut into 12 slices covering the holocomplex (slice 1) and subcomplexes of different sizes (slices 2–12; Fig. 5e ). The protein content in each slice was determined by spectral counting-based label-free semiquantitative proteomics ( Supplementary Tables 4–7 ). We quantified 36 of the 44 complex I subunits (plus NDUFA4, which has now been identified as a complex IV subunit [14] ). We compared C57Bl/6 and ICRFa mice at 8 months of age as well as AL and DR C57Bl/6 mice at 15 months of age (following 12 months of DR) with three mice analysed separately per group. Peptide counts of the various proteins making up the holoenzyme were widely different, even after normalization for total peptide counts per mouse ( Supplementary Tables 4–7 ). The detection efficiency in the major (holocomplex) slice in our proteomic approach is similar to other recent proteome profiling approaches [13] , [14] . Importantly, our counts were highly reproducible between experiments and mice with an average standard error below 15% ( Supplementary Tables 4–7 ). Relative amounts of all complex I proteins that were detected in subcomplexes are shown in the heatmaps ( Fig. 5f–i ) assuming equimolar stoichiometry in the holocomplex. It should be noted that equimolar stoichiometry in the mammalian complex I holocomplex has so far been proven for only 7 out of 14 tested complex I subunits [12] , therefore, absolute quantification should not be attempted from these data. Our results indicate that complex I subunits NDUFA7, 10 and 12 are exclusively found in smaller (below 200 kDa) subcomplexes (and in the holocomplex), whereas most other subunits are preferentially located in larger complexes (>500 kDa). Importantly, comparisons between the treatments show less matrix subunits in subcomplexes in mice treated with DR (compare Fig. 5g,f ) and in ICRFa ( Fig. 5i ) versus C57Bl/6 ( Fig. 5h ) mice at the same age. In fact, hardly any complex I subcomplexes could be found in 8-month-old ICRFa mice ( Fig. 5i ). Moreover, a comparison between C57Bl/6 mice under AL feeding shows increased accumulation of subcomplexes from 8 months ( Fig. 5h ) to 15 months ( Fig. 5f ) of age. Taken together, these experiments suggest that complex I in liver mitochondria is more efficiently assembled in long-living mice, and this is counteracted by increasing age. Less efficient complex I assembly increases ROS and senescence The catalytic subunits of complex I are located in the matrix arm, but proton pumping occurs via the membrane arm; hence the electron transfer to the Q-pool is only possible with the fully assembled complex I. ‘Superfluous’ matrix subunits may produce superoxide on its own [15] without involving electron transfer activity in the ETC. We hypothesized that less complete assembly of complex I should result in less efficient electron transfer and oxidative pohsphorylation (OXPHOS)-dependent ATP production per unit of substrate used, and higher ROS production. To test this hypothesis, we disrupted the complex I assembly by small interfering RNA (siRNA)-mediated gene silencing of the complex I assembly factor NDUFAF1 in HeLa cells ( Fig. 6a ), which increases the relative abundance of partially assembled complex I [16] , decreasing protein abundance and activity in the holocomplex ( Fig. 6f ). Reduction of NDUFAF1 protein abundance to <50% was not associated with changes in the amount of the complex II protein SDHA, but with a potentially compensatory increase of PhB ( Fig. 6a ). This was associated with lower oligomycin-sensitive oxygen consumption and higher basal acidification rates in the medium ( Supplementary Fig. 6 ), resulting in lower mitochondrial OXPHOS and higher glycolytic ATP production ( Fig. 6b ). Furthermore, despite lower basal oxygen consumption rates ( Supplementary Fig. 6 ), mitochondrial superoxide production was increased as measured by fluorescence intensity of MitoSOX, a dihydroethidine (DHE) derivative directed into mitochondria ( Fig. 6c ). Fluorescence of the pan-cellular superoxide-sensitive dye DHE was slightly but significantly increased, and hydrogen peroxide release from complex I in isolated HeLa cell mitochondria under basal conditions was also increased following NDUFAF1 knockdown, with a tendency to increased H 2 O 2 release under maximum stimulated respiration as well ( Fig. 6d ). However, dihydrorhodamine-123 (DHR-123) fluorescence indicating cellular peroxide levels was unchanged ( Fig. 6c ), which might indicate that under the given experimental conditions in HeLa cells hydrogen peroxide was still efficiently detoxified by cytoplasmic antioxidants. Together, these data indicate that mitochondrial superoxide production increased despite of lower OXPHOS activity as a result of NDUFAF1 knockdown. 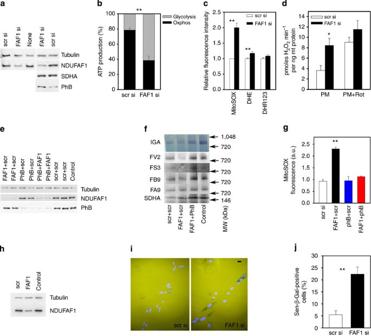Figure 6: Knockdown of the complex I assembly factor NDUFAF1 increases mitochondrial ROS production and induces cellular senescence. (a) Western blots of the indicated proteins in HeLa cells treated with scrambled siRNA (scr si), siRNA against NDUFAF1 (FAF1 si) or untreated. (b) Relative ATP production by glycolysis (grey) and oxidative phosphorylation (black) in HeLa cells treated with the indicated siRNAs. Data are mean±s.e.m.,n=3, **P<0.001,t-test. (c) Relative fluorescence intensity of the ROS indicator dyes MitoSOX, dihydroethidine (DHE) and dihydrorhodamine-123 (DHR-123) in HeLa cells treated as indicated. Data are mean±s.e.m.,n=6, **P<0.001,t-test. (d) H2O2release under pyruvate+malate (native conditions) and under PM+rotenone (CI max). Data are mean±s.e.m.,n=3, *P<0.05,t-test. (e) Western blots of the indicated proteins in HeLa cells treated with siRNAs in the indicated combinations. (f) Complex I in-gel activity (IGA) and BN/western for the complex I matrix arm subunits NDUFV2 and NDUFS3, the membrane arm subunits NDUFA9 and NDUFB9 and for SDHA as loading control. HeLa cells were treated with the indicated combinations of siRNAs. Bands at the level of the holocomplex I or complex II (SDHA), respectively, are shown. (g) Mitochondrial superoxide production (MitoSOX fluorescence activity) in HeLa cells treated with the indicated combinations of siRNAs. Data are mean±s.e.m.,n=4, **P<0.001, analysis of variance. (h) Western blots of NDUFAF1 and tubulin (control) in MRC5 human fibroblasts treated with siRNAs as indicated. The bar indicates 25 μm. (i) MRC5 fibroblasts treated with scr si (left) or NDUFAF1 siRNA (right) and stained for Sen-β-Gal (dark blue cytoplasmic stain). Nuclei are counterstained with DAPI. (j) Fractions of Sen-β-Gal-positive MRC5 cells following transfection with either scr si or anti-NDUFAF1 siRNA. Data are mean±s.e.m.,n=6. **P<0.001, Student’st-test. Figure 6: Knockdown of the complex I assembly factor NDUFAF1 increases mitochondrial ROS production and induces cellular senescence. ( a ) Western blots of the indicated proteins in HeLa cells treated with scrambled siRNA (scr si), siRNA against NDUFAF1 (FAF1 si) or untreated. ( b ) Relative ATP production by glycolysis (grey) and oxidative phosphorylation (black) in HeLa cells treated with the indicated siRNAs. Data are mean±s.e.m., n =3, ** P <0.001, t -test. ( c ) Relative fluorescence intensity of the ROS indicator dyes MitoSOX, dihydroethidine (DHE) and dihydrorhodamine-123 (DHR-123) in HeLa cells treated as indicated. Data are mean±s.e.m., n =6, ** P <0.001, t -test. ( d ) H 2 O 2 release under pyruvate+malate (native conditions) and under PM+rotenone (CI max). Data are mean±s.e.m., n =3, * P <0.05, t -test. ( e ) Western blots of the indicated proteins in HeLa cells treated with siRNAs in the indicated combinations. ( f ) Complex I in-gel activity (IGA) and BN/western for the complex I matrix arm subunits NDUFV2 and NDUFS3, the membrane arm subunits NDUFA9 and NDUFB9 and for SDHA as loading control. HeLa cells were treated with the indicated combinations of siRNAs. Bands at the level of the holocomplex I or complex II (SDHA), respectively, are shown. ( g ) Mitochondrial superoxide production (MitoSOX fluorescence activity) in HeLa cells treated with the indicated combinations of siRNAs. Data are mean±s.e.m., n =4, ** P <0.001, analysis of variance. ( h ) Western blots of NDUFAF1 and tubulin (control) in MRC5 human fibroblasts treated with siRNAs as indicated. The bar indicates 25 μm. ( i ) MRC5 fibroblasts treated with scr si (left) or NDUFAF1 siRNA (right) and stained for Sen-β-Gal (dark blue cytoplasmic stain). Nuclei are counterstained with DAPI. ( j ) Fractions of Sen-β-Gal-positive MRC5 cells following transfection with either scr si or anti-NDUFAF1 siRNA. Data are mean±s.e.m., n =6. ** P <0.001, Student’s t -test. Full size image PhBs may act as chaperones for incompletely assembled complex I subunits. To test this idea, we performed double knockdowns for NDUFAF1 and PhB in HeLa cells ( Fig. 6e ; see Supplementary Fig. 7 for uncropped scans). NDUFAF1 knockdown alone reduced activity of the fully assembled complex I ( Fig. 6f ) as described before [16] . It also decreased protein abundance in the holocomplex with a preference for matrix arm proteins ( Fig. 6f ). Importantly, both activity and protein abundance were restored by additional siRNA-mediated suppression of PhB ( Fig. 6f ). Moreover, knockdown of PhB completely rescued the increase in mitochondrial superoxide in NDUFAF1 KD cells ( Fig. 6g ). It also tended to rescue hydrogen peroxide release from isolated HeLa mitochondria under conditions of maximum ROS production ( Supplementary Fig. 8 ). Finally, we asked the question whether disruption of complex I assembly would induce somatic cell ageing. When NDUFAF1 was reduced by siRNA-mediated knockdown in primary human MRC5 fibroblasts ( Fig. 6h ; see Supplementary Fig. 9 for uncropped scans ), cell growth was decelerated and cells became positive for senescence (Sen)-associated β-galactosidase ( Fig. 6i ), an established marker for cell senescence [17] . The increase in the frequency of Sen-β-Gal-positive cells was highly significant ( Fig. 6j ), indicating that disturbance of complex I assembly induced premature senescence of normal somatic cells. Few earlier studies examined changes in the liver mitochondrial proteome between young, old and dietary restricted animals. These identified a low number of ETC subunits, generally at lower abundance under DR and increased in old animals [18] , [19] , [20] , which is consistent with our data. Similar results were found in other tissues including skeletal muscle [21] and heart [22] , [23] , although Ghosh et al. [24] reported that ageing reduced some ETC subunits along with decreased ROS production in human skeletal mitochondria. In-depth interpretation of many of these studies has been hampered by low coverage and/or sensitivity. We focused on changes that occur in the mitochondrial proteome of long-living animals at an early age and thus might be causally involved in longevity. We chose two models of longevity: DR, which leads to a robust extension of lifespan in our C57Bl/6 mice [25] , and comparison between two strains (C57Bl/6 and ICRFa). We used a gel-free quantitative proteomics approach enabling detection of a large fraction of the mitochondrial proteins without recognizable bias against hydrophobic polypeptides. Use of a novel Bayesian model to evaluate the significance of differences in protein abundance from the measured peptide label distributions [26] allowed high confidence even in relatively small fold-changes in protein abundance. Although we were aware of issues with the accuracy of relative quantification owing to signal compression effects when using isobaric approaches such as TMT [27] , these do not affect our conclusions as they are based on high-confidence protein abundance changes, not on their magnitude. Critically, what was common in long-lived animals was the low abundance of many of the ETC subunits proteins at a young age, which was reversed at old age. Downregulation of individual components of the ETC has been found to extend lifespan in Podospora anserina [28] , Caenorhabditis elegans [29] , [30] and Drosophila melanogaster [31] , and resulted in lower acceleration of mortality with age in mice [32] . In these models, successful lifespan extension was often ascribed to induction of stress–response pathways, specifically the mitochondrial unfolded protein response [33] , [34] , although we did not see evidence for it in our long-living mice. Our data suggest that a coordinated decrease of ETC protein abundance, as found in the mitochondria from long-living mice, does not necessarily compromise mitochondrial function, so far as it supports efficient complex (and, possibly, ETC supercomplex) formation. In fact, emerging data indicate close interactions among supercomplex formation, ETC stability and ETC functionality, showing that supercomplex destabilization might contribute to increased ROS production during ageing [35] . Our study identified low abundance of complex I matrix arm subunits as the common feature in multiple tissues and multiple intervention models in long-living mice. Recent metabolic labelling study in mice [5] showed that matrix arm proteins had shorter half-lives than membrane arm proteins in liver and heart, which is in agreement with the idea that matrix arm proteins might exist to a larger extent as free monomers or in less stable, smaller complexes. Furthermore, Lambert et al. [36] identified low complex I content as the most probable explanation of the low hydrogen peroxide release in pigeon heart mitochondria as compared with the mouse. Our data specify this result by correlating the abundance of complex I matrix subunits with ROS production. The structure of the mammalian complex I holocomplex is still far from clear [37] . So far, stoichiometric relationships have only been established for 7 out of the 44 subunits in the holoenzyme [12] . However, at least in HEK293 cells, the majority of complex I subunits exists in a steady-state equilibrium between supercomplexes, the holocomplex and subcomplexes [12] , [13] . Our data confirm this finding for mitochondria in mouse liver. Importantly, we show that lower amounts of matrix arm subunits in mitochondria from long-lived mice are associated with a shift in the equilibrium from subcomplexes towards the holocomplex, suggesting that the relative abundance of the matrix subunits is a particularly important factor for functional optimization through more complete complex I assembly status. Based on our data, we propose the following model ( Fig. 7 ): relatively low abundance of matrix arm subunits favours more complete assembly of complex I. This enables efficient use of substrate for proton pumping and electron transport, resulting in high efficacy of ATP generation and only obligatory levels of superoxide production during normal electron transfer. It might be an adaptation to DR or other longevity-enabling intervention, which is independent from proton leak-mediated regulation of efficacy of ATP synthesis, and is associated with limited ROS production and long lifespan ( Fig. 7 , left). There are various possible mechanisms linking complex I assembly and activity with ROS production. For instance, an inverse relationship between complex I activity and ROS production was found in fibroblasts from patients with inherited complex I disorders [38] . This might be because of an impact of complex I activity onto the local redox balance via oxidation of the NAD/NADH pool. Alternatively, severely compromised complex I activity with defective proton pumping might be linked to compensatory ATP hydrolysis by ATP synthase, resulting in high mitochondrial membrane potential causing high ROS production through reverse-electron flow at complex I [39] . However, such an inverse correlation between complex I activity and ROS production is far from universal: In many cross-species comparisons and in multiple DR experiments, lower mitochondrial superoxide production in long-living cohorts was associated with a lower or unchanged complex I activity [40] , [41] , [42] , [43] . Our model ( Fig. 7 ) might explain this apparent paradox. 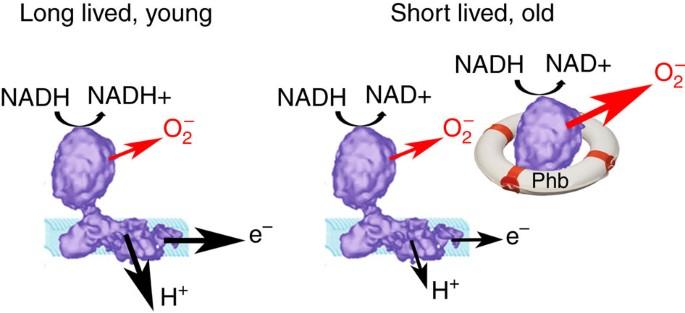Figure 7: Non-assembled catalytic matrix arm subunits cause decreased electron transport and increased ROS production. If complex I is fully assembled, ROS production is minimum, substrate is used for efficient proton pumping and electron transport, and this is associated with longevity (left). Incompletely assembled matrix arm subunits (which might be stabilized by PhB) can still use substrate and produce superoxide, but without proton pumping or electron transport, thus reducing the overall efficiency of the ETC and increasing superoxide output (right). Figure 7: Non-assembled catalytic matrix arm subunits cause decreased electron transport and increased ROS production. If complex I is fully assembled, ROS production is minimum, substrate is used for efficient proton pumping and electron transport, and this is associated with longevity (left). Incompletely assembled matrix arm subunits (which might be stabilized by PhB) can still use substrate and produce superoxide, but without proton pumping or electron transport, thus reducing the overall efficiency of the ETC and increasing superoxide output (right). Full size image In old and/or shorter living mice, the relative amounts of complex I matrix arm subunits are increased, which might be caused by excessive production or insufficient degradation of unassembled matrix arm subunits, or by low efficacy of complex I assembly, although, complex I assembly factors NDUFAF1 and Acad9 were of equal abundance in all mice ( Supplementary Data 1 ). The fact that abundance of the chaperone complex, PhB, changed in parallel to that of complex I matrix arm subunits ( Supplementary Table 1 ), makes stabilization of unassembled subunits as its function an attractive possibility ( Fig. 7 , right). This was confirmed by our data showing that PhB knockdown rescued complex I formation and the enhanced complex I-dependent ROS production in cells with compromised complex I assembly. It is interesting in this context that diminished expression of PhBs is associated with pathological conditions such as chronic obstructive pulmonary disease [44] , whereas increased expression of PhBs was associated with oxidative stress [45] . Importantly, PhB depletion increased lifespan in C. elegans mutants with compromised ETC [46] , thereby suggesting possible long-term deleterious effects of chaperone-mediated stabilization of individual ETC components. Partially assembled subcomplexes of complex I can produce superoxide on their own [15] but cannot contribute to electron transfer and proton pumping, diminishing the efficiency of substrate utilization ( Fig. 7 , right). Such a state might be termed ‘mitochondrial cachexia’. This model might be applicable to a number of mitochondrial diseases that are caused by mutations in complex I assembly factors. Cells from these patients accumulate partially assembled complex I subcomplexes and show impaired mitochondrial oxygen consumption [47] . Moreover, aggressiveness of breast tumour cells in humans has been associated with a high ratio of matrix (NDUFS3) to membrane subunits (NDUFB9) of complex I [48] . According to our results, high NDUFS3/NDUFB9 ratios are indicative of suboptimal complex I assembly, which is in turn associated with a shift in ATP production from oxidative phosphorylation towards glycolysis ( Fig. 6 ). Defective complex I assembly, or generally an imbalance between different subunits of the ETC, might thus be a mechanistic cause of shifts in the energy production that has been linked to fast growth and aggressiveness of tumour cells [49] . Moreover, unbalanced complex I assembly might cause premature cellular senescence by either increased ROS production inducing DNA damage, including premature telomere shortening [50] , [51] , [52] , by changed energy metabolism [53] , or both. Cell senescence is mechanistically linked to accelerated ageing: Senescent cells increase with age in multiple tissues of mice [54] and primates [55] and decrease in frequency under DR [56] . They secrete bioactive molecules including cytokines [57] and ROS [58] that can damage neighbouring cells [59] . Targeted ablation of senescent cells rescued age-related functional deterioration in multiple tissues in at least one progeroid mouse model [60] . Together, these data provide a mechanistic link between mitochondrial complex I homeostasis, cell senescence and organism ageing. In conclusion, our data suggest the intriguing possibility that differences in the ratio of matrix to membrane subunits and the completeness of the assembly of complex I could contribute to more efficient regulation of the energy producing machinery that in turn limits excessive ROS production by complex I and enables enhanced longevity. This might lead to novel intervention approaches in areas as different as sarcopenia, oncology or frailty. Mice C57Bl/6 male mice were purchased from Harlan (Blackthorn, UK) or (for the rapamycin experiment) backcrossed from TERC+/− mice (strain B6.Cg-Terc tm1Rdp /J, Jackson Laboratories). ICRFa are a substrain of C57Bl/6 (ref. 7 ) kept as a long-established ageing colony at Newcastle. Male mice were housed [25] in cages (56 cm × 38 cm × 18 cm, North Kent Plastics, Kent, UK) of groups of 4–6 that did not change from weaning. Mice were provided with saw dust and paper bedding and had AL access to water. Mice were housed at 20±2 C under a 12-h light/12-h dark photoperiod with lights on at 7:00 am. Group sizes for lifespan experiments were (censored events in brackets): C57Bl/6 AL 310 (172), C57Bl/6 DR 241 (157) and ICRFa 2391 (1,061). DR at 60% of AL intake was initiated at 3 months of age and lasted for either 5 or 12 months. DR at 60% of AL intake was initiated at 3 months of age and lasted for either 5 or 12 months. For the rapamycin experiment, control chow was supplemented with 0.067 mg of rapamycin per day per mouse [10] , [61] (gift from John Strong, TX, USA). All work complied with the guiding principles for the care and use of laboratory animals and was licensed by the UK Home Office (PPL60/3864). Mitochondrial isolation Mouse liver was chopped and rinsed in ice-cold isolation medium (250 mM sucrose, 5 mM Tris Base and 2 mM EGTA, pH 7.4, at 4 °C), and was homogenized by a glass homogenizer (Wheaton 15 ml Dounce tissue grinder) using six strokes with a loose-fit pestle and centrifuged at 1,050 g for 3 min. The supernatant was centrifuged at 11,630 g for 10 min, and the pellet was washed two more times in isolation medium. The resultant pellet was resuspended in 0.5 ml of isolation medium (crude mitochondria) followed by purification by Percoll density centrifugation using a stepwise density gradient of 2 ml 80%, 6 ml 52% and 6 ml 26% Percoll in isolation medium, at 41,100 g for 45 min. The mitochondria were collected from the 26%/52% interface and washed twice with isolation medium at 11,600 g to obtain the purified mitochondria [62] . Mouse brain mitochondria were isolated from whole brain. The brain was removed and put in ice-cold isolation medium (250 mM sucrose, 10 mM Tris base and 0.5 mM EDTA, pH 7.4, at 4 °C ) as quickly as possible after the mouse was killed, homogenized using a glass homogenizer (Wheaton 15 ml Dounce tissue grinder) with eight strokes with a loose-fitting pestle and centrifuged at 2,000 g for 3 min. The supernatant was collected and centrifuged at 12,500 g for 10 min to obtain the pellet. The pellet was resuspended in 3% Ficoll solution (diluted from 6% Ficoll solution with water) and carefully layered onto the 6% Ficoll solution (240 mM mannitol, 60 mM sucrose, 50 μM EDTA and 10 mM Tris base, pH 7.4 °C, with 6% (w/w) Ficoll) and centrifuged at 11,500 g for 15 min. The supernatant was sharply decanted and the loose, fluffy top layer of the pellet was removed. The resultant pellet was resuspended with isolation medium and centrifuged at 11,500 g for 10 min to obtain the mitochondrial pellet [4] . Mitochondria from HeLa cells were isolated using a mitochondrial isolation kit (MACS Miltenyi Biotec) according to the manufacturer’s instructions. Mitochondrial proteomics by TMT labelling. Frozen mitochondrial pellets were disrupted by three cycles of thawing on ice and refreezing in liquid N 2 . Subsequently, 150 μg protein per sample were dissolved in 50 μl of 1.5 M urea and 90 mM triethylammonium bicarbonate, pH 8. Samples were reduced with 5 μl of 200 mM Tris(2-carboxyethyl)phosphine in 50 mM triethylammonium bicarbonate at 55 °C for 1 h, followed by the addition of 5 μl of 375 mM iodoacetamide (AppliChem) and incubation for 30 min at room temperature in the dark. Proteins were digested with trypsin (1:50 w/w) overnight. Peptides were labelled with 6-plex Tandem Mass Tags (TMT) (Pierce, Cramlington, UK) according to manufacturer’s instructions. Samples were analysed in two sets of experiments (Expt1 and Expt2), each containing one-pooled sample for cross-standardization. In addition to the pool sample, Expt1 consisted of 3 × DR and 2 × AL C57/Bl6 and Expt2 included 2 × young ICRFa, 2 × old ICRFa and 1 × AL C57/Bl6. Every experimental sample was from one separate animal. Samples were separated into 11 (Expt1) or 10 (Expt2) fractions using a 3100 Offgel fractionator (Agilent) following the manufacturer’s instructions. Peptides from each fraction were analysed on Dionex Ultimate 3000 nano-HPLC system with a Dionex PepMap column (75 μm × 250 mm) coupled to an Orbitrap LTQ XL mass spectrometer. Peptides were eluted with a gradient from 5% acetonitrile (MeCN), 0.08% formic acid to 60% MeCN, 0.08% formic acid over 132 min. The capillary voltage was set to 200 °C and the spray voltage to 1.6 kV. Survey scans were acquired in the Orbitrap with a resolution of 30,000 at m/z 400 Da. Up to three sets of data-dependent MSMS scans were acquired for the three most intense precursor ions, with a collision-induced dissociation (CID) spectrum (in the LTQ) and an higher energy collision dissociation (HCD) spectrum (in the Orbitrap) triggered for the same precursor. CID was performed with a target value of 10,000 in the linear ion trap, collision energy of 35%, Q value of 0.25 and an activation time of 30 ms. HCD spectra were acquired with a resolution of 7,500 (at m/z 400) and a collision energy of 60%. Raw data were processed using ProteomeDiscoverer v 1.1 (Thermo). HCD spectra were used for the ‘reporter ions quantizer’ node using an integration window tolerance of 20 p.p.m. and TMT batch-specific isotope impurity correction factors and raw quan values as an output variable. Using Proteome Discoverer as an interface, a concatenated database containing mouse proteins from swissprot (v 2010_04), trembl (v 2010_04) and cRAP ( ftp://ftp.thegpm.org/fasta/cRAP ), containing a total of 55,309 sequences, was searched with the CID and the HCD spectra using Mascot v. 2.2 (Matrix Science) and the following parameters: 1 missed tryptic cleavage site, 1% FDR (determined using a reversed decoy database), 10 p.p.m. precursor tolerance, 0.8 Da fragment ion tolerance, carbamidomethyl (on Cys) and 6-plex TMT (on N-termini and on Lys) as fixed modifications, oxidation (Met), deamidation (Gln and Asn), acetylation (Lys) and pyro-Glu as variable modifications. Quantitation and identification results were exported together as tsv files. Using an in-house written script, these files were then converted into a format that was suitable for processing by the purpose-written Bayesian tool dpeaqms (deposited on R-forge, http://r-forge.r-project.org/projects/dpeaqms/ ). Dpeaqms [26] uses a Bayesian approach and Markov Chain Monte Carlo methods to calculate the posterior probability β that the conducted experiments indicate a systematic change in protein concentration between groups. The statistical model takes into account (i) a sample specific normalization term (to account for loading differences); (ii) a mean reporter ion intensity (assuming no systematic differences) for an MSMS spectrum; (iii) the mean difference in log intensity in which a systematic difference between a sample’s group and the reference group is observed; and (iv) independent and identically distributed noise terms following a normal distribution. A β ≥0.5 was chosen as threshold for different abundance, accepting a FDR in the order of 1% (ref. 26 ). To perform group comparisons across both experiments, that is, for the DR–AL and the ICRFa–C57Bl/6 comparisons, pooled samples were used as a standard (combined analysis). A DR–AL comparison was also performed within Expt1 only, and the young–old comparison was only made in Expt2. For these comparisons, the data were analysed within the set and the pooled sample was not used (solo analyses). In the DR–AL comparison, there were 139 and 141proteins significantly different in abundance using combined or solo analysis, respectively. Calculated β values and fold changes were very similar for most of the proteins. Only 10 proteins were found altered in the solo analysis but not in the combined one, and eight proteins were altered in the combined analysis but not in the solo analysis ( Supplementary Table 1A ). This validates our use of pooled samples as a standard and indicates that the chosen number of animals are sufficient for a robust estimate of differences. For the final DR–AL comparison, we considered proteins as confidently different in abundance only when their β values were ≥0.5 in both sets of analysis. The results for all the comparisons are presented as Supplementary Data 1 . For mitochondria-specific KEGG pathway enrichment analysis, KEGG pathway finder was used to identify all KEGG pathways that contain at least one mitochondrial protein that has changed with a probability β >0.5. Next, all mitochondrial proteins belonging to each identified KEGG pathway were identified using MitoMiner v2 (ref. 8 ). KEGG pathway terms enrichment analysis was performed in R with a hypergeometric distribution function separately for proteins that were either more or less abundant under DR. This was compared with enrichment of the same pathways based on proteins more or less abundant, respectively, in young or old ICRFa. Heatmaps of the ETC subunits were drawn using Cytoscape. Mitochondrial complex I profiling Mitochondria were solubilized in sample buffer (50 mM BisTris, 6 N HCl and 50 mM NaCl, 10% w/v glycerol, pH 7.2) with detergent dodecylmaltoside at 3.2 g/g (detergent/protein) ratio. The samples were separated by BN gel electrophoresis according to manufacturer’s instructions (Life Technologies), using a 4–16% gel. Gel lanes were cut into 12 slices ( Fig. 4e ), which were destained, reduced using 10 mM Dithiothreitol (AppliChem) and alkylated in the dark using 50 mM iodoacetamide (AppliChem before digestion with trypsin (Promega) for 18 h. The digested peptides were extracted from the gel pieces, desalted using stage tips [63] , concentrated in a speedvac and acidified using 1% trifluoroacetic acid. Peptides were separated using a PepMap column (250 mm × 75 μm, Thermo) and a water/acetonitrile gradient from 4–40% acetonitrile over 100 min. A combination of data from preliminary experiments and gpmdb [64] was used to generate an accurate mass inclusion list [65] in XCalibur. Peptide retention times in the inclusion lists were either obtained from our own experimental data or estimated using the pyteomics python framework. Precursor ions were detected in positive mode at 350–1,600 m/z with a resolution of 60,000 (at 400 m/z) and a fill target of 500,000 ions and a lockmass was set to 445.120023, m/z. The six most intense ions of the inclusion list (with a target value of 1,000 ions) followed by the four most intense other ions (also with a target value of 1,000 ions) in each MS scan were isolated, fragmented using CID and a normalized collision energy of 35 eV and measured in the linear ion trap. Peaklists in the Mascot generic format (*.mgf) were generated using msconvert (proteowizard.sourceforge.net) [66] and the mouse proteome (ensembl NCBI 37.64) was searched using an in-house installation of X!Tandem with the gpm interface [67] (version 2013.09.01.1) and carbamidomethylation set as a fixed modification, methionine oxidation as a variable modification. Two refinement steps were included in the search to include deamidation and methylation artefacts occurring in the gel. The protein level false-positive rate (as defined in: http://wiki.thegpm.org/wiki/False_positive_rate ) for all searches was <1%. BioML files obtained from X!Tandem were parsed and the results were annotated using in-house written python scripts (available from the authors upon request). Peptide and protein sequences were extracted, annotated with band position, repeat number (1–3) and experimental treatment, peptide lists were filtered to include only complex I peptides, PhB and NDUFA4 and rolled up into protein lists. The number of peptides found for each protein in each band was normalized by dividing it by the number of all identified peptides for the corresponding lane (mitochondrial sample) in the BN gel and then multiplied with 10 6 . Normalized peptide counts were averaged over three mice per group analysed independently. Averaged counts were used to generate heatmaps following normalization to counts in slice 1 (the holocomplex). Functional experiments Mitochondrial oxygen consumption rates were measured using Seahorse XF 24 analyzer according to the manufacturer’s instructions (see also ref. 68 and comments therein). Five micrograms per well mitochondria were attached to the 24-well plate by centrifugation (2,500 g for 10 min at 4 °C), and oxygen consumption rates were measured in the assay buffer (115 mM KCl, 10 mM KH 2 PO 4 , 2 mM MgCl 2 , 3 mM HEPES, 1 mM EGTA and 0.2% fatty acid-free BSA, pH 7.2, at 37 °C) with substrate (5 mM pyruvate and 5 mM malate for complex I-linked substrate or 4 mM succinate for complex II-linked substrate). State 3 oxygen consumption rates were obtained by adding 4 mM ADP. Mitochondrial hydrogen peroxide release was measured fluorometrically in the presence of exogenous superoxide dismutase (15 U μl −1 ), horseradish peroxidise (2 U ml −1 ) and Amplex red (50 μM) at 37 °C, and the fluorescence signals were calibrated against a hydrogen peroxide standard. Western blots and BN gel For SDS–PAGE experiments, 20 μg of mitochondrial proteins or 15 μg of whole-cell extracts were loaded in 15% SDS gels. Membranes were probed with the following antibodies: NDUFA9 (1:1,000, Abcam, ab14713), NDUFAF1 (1:10,000, Abcam, ab79826), NDUFS3 (1:1,000, Abcam, ab110246), NDUFB9 (1:1,000, Abcam, ab106699), NDUFV2 (1:1,000, Proteintech, 15301-1-AP), PhB (1:1,000, Abcam, ab28172), SDHA (1:1,000, Abcam, ab14715), UQCRC2 (1:1,000, Abcam, ab14745) and tubulin (1:1,000, Cell Signaling, no. 21485). Proteins separated by BN PAGE were transferred to Polyvinylidene fluoride (PVDF) membranes and western blotting was performed as above. Alternatively, the BN gels were used for in-gel activity assays for complex I by incubating the gel in the assay buffer consisting of 5 mM Tris/HCl with 2.5 mg ml −1 nitrotetrazolium blue and 0.1 mg ml −1 NADH (pH 7.4). Cell transfection experiments Subconfluent cultures of HeLa or MRC5 cells were treated with 10 nM each of anti-NDUFAF1 siRNA (Qiagen, SI04312413, Hs_NDUFAF1_9), anti-PHB siRNA (Qiagen, SI00301175, Hs_PHB_6) or control siRNA (Qiagen, cat. no. 1027281) in various combinations. Seventy-two hours after the transfection, cells were stained using either 10 μM DHE, 10 μM DHR-123 or 1 μM MitoSox, and ROS levels were measured by flow cytometry [52] . Cellular oxygen consumption and media acidification rates were measured in a Seahorse XF24 analyzer with sequential injections of oligomycin (0.5 μM), Carbonyl cyanide 4-(trifluoromethoxy)phenylhydrazone (FCCP) (2.5 μM), Rotenone (0.5 μM) and Antimycin (2.5 μM). ATP production rates were calculated according to ref. 69 . MRC5 human fibroblasts were triple transfected at 4–5 day intervals during which their growth rate was monitored. Cells were stained for Sen-β-Gal activity at 23 days after the first transfection as described [17] , [58] . Accession codes The mass spectrometry proteomics data have been deposited in the Proteomics Identifications database (PRIDE) under the accession code PXD000272 How to cite this article: Miwa, S. et al. Low abundance of the matrix arm of complex I in mitochondria predicts longevity in mice. Nat. Commun. 5:3837 doi: 10.1038/ncomms4837 (2014).